Automated long-term tracking and social behavioural phenotyping of animal colonies within a semi-natural environment Social behaviour has a key role in animal survival across species, ranging from insects to primates and humans. However, the biological mechanisms driving natural interactions between multiple animals, over long-term periods, are poorly studied and remain elusive. Rigorous and objective quantification of behavioural parameters within a group poses a major challenge as it requires simultaneous monitoring of the positions of several individuals and comprehensive consideration of many complex factors. Automatic tracking and phenotyping of interacting animals could thus overcome the limitations of manual tracking methods. Here we report a broadly applicable system that automatically tracks the locations of multiple, uniquely identified animals, such as mice, within a semi-natural setting. The system combines video and radio frequency identified tracking data to obtain detailed behavioural profiles of both individuals and groups. We demonstrate the usefulness of these data in characterizing individual phenotypes, interactions between pairs and the collective social organization of groups. Social interaction and communication are basic complex behavioural features crucial to the survival of all animal organisms in their ecosystems. Laboratory animals, from mouse and rat to simpler animal models, such as fruit fly, display a wide range of social behaviours that can be quantitatively measured with laboratory techniques [1] , [2] . Indeed, the study of animal social behaviours in laboratory settings has tremendous impact on a wide range of research fields, including psychology, ecology, evolution, genetics and neuroscience. Furthermore, there is increasing recognition in the importance of defining the molecular and neuronal principles of social interactions that could facilitate the understanding and treatment of social-related symptoms as are observed in many common neuropsychiatric disorders (for example, autism and schizophrenia) [1] , [3] . Successful social behaviour analysis requires recognition of key social interactions in a realistic context that captures social and environmental situations that occur in natural habitats [4] . However, the increasing number of methods developed to study animal social behaviour within laboratory environments [1] , [3] typically achieve reliability by forsaking environmental complexity. This is largely because studying the social behaviour of groups for extended periods of time and within semi-natural environments is a highly challenging task. It requires the tracking of multiple identified individuals with a high spatiotemporal precision that can allow for accurate identification of a complex series of behavioural patterns. Manual quantification of such behavioural traits requires a vast time investment in terms of both training and analysis, while remaining susceptible to errors and subjectivity, and potentially overlooking the most meaningful phenotypes [5] , [6] , [7] . To circumvent inherent human constraints, there is a critical need for machine-based tracking and behavioural phenotyping technologies that are applicable toward the analysis of socially interacting groups of animals. Several research teams have developed automated vision-based tracking tools that support behavioural phenotyping of a single individual in its home cage [8] , [9] , [10] , a pair of socially interacting animals [11] , [12] , [13] , [14] and of individuals in the context of large groups [15] , [16] , [17] . However, such methods limit: (i) the number of animals that can be concurrently observed over an extended period of time (for example, up to three mice) and (ii) the size of the testing environments, alongside a requirement for minimal visual obstructions. Techniques for tracking large numbers of targets (for example, humans) moving in a crowded environment usually rely on detection of distinguishable vision-based physical features for each tracked individual [18] . However, such tracking solutions cannot be translated to analysis of small species that exhibit very few differences in shape, size and colour, such as in most rodents, fish and insects. Radio-frequency identified (RFID) tagging has been successfully applied to track the position of uniquely identified animals within a group [19] , [20] . RFID technology allows for remote identification of objects that bear specific vision-independent tag (small glass-coated transponders labelling), which transmit information to antenna receivers. This technology supports unique tagging and tracking of an indefinite number of individuals, which can be monitored for unlimited periods. Although RFID-based animal-tracking solutions efficiently follow the gross movements of large numbers of animals in both field and laboratory conditions, they have rarely been applied to evaluate rodent social behaviour. This is probably due to their low spatial accuracy (usually greater than 20–40 cm) and relatively low temporal resolution [20] , [21] , [22] , [23] , [24] , [25] , which fails to generate high-precision tracking of animals moving at moderate to high speed, as in the case of small rodents (for example, mouse maximum velocity can exceed 110 cm s −1 (ref. 26 )). Here we describe an automatic behavioural analysis of multiple socially interacting animals, such as small rodents, within diverse complex environments and social contexts, and over testing durations of several minutes up to several weeks (limited only by data storage capacity). The method simultaneously and continuously tracks the identity and spatial position of many animals (for example, ≥10 mice), without the need for visual tagging, by integrating video and RFID tracking data sets, which are time-synchronized and then fused by means of a machine-based algorithm. This hybrid-tracking method simultaneously provides X , Y coordinates position, speed and orientation of numerous uniquely identified socially interacting individuals, with a mean spatial precision of ~±0.5 cm and a temporal precision of ~30 ms ( Supplementary Movie 1 , Fig. 1a ). Our technique allows for the evaluation of the effects of group characteristics on individual behavioural traits (such as, locomotion pattern; Supplementary Movie 2 ). Furthermore, the tracking technology constitutes a useful tool toward the definition of complex social interactions between multiple pairs of animals, as well as in the analysis of the formation and stability of dominant-subordinate hierarchy within a group ( Supplementary Movie 3 , Fig. 1c ). 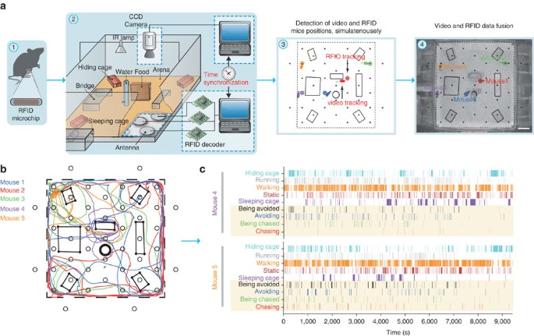Figure 1: Automated behavioural phenotyping system for multiple individually identifiable socially interacting animals. (a) Presentation of the major system components and operational stages to capture theX–Ycoordinates and identification of each animal in the arena, for each processed frame. (1) Before its introduction to the enclosure, two RFID microchips (~2 mm in diameter, ~10 mm in length) are subcutaneously implanted in the ventral part of the front and hind foot of each tested animal. (2) The RFID-tagged animals are placed in a semi-natural enclosure equipped with a large central exploratory arena and eight peripheral sleeping nests. Time-synchronized video and RFID-tracking systems are used to survey the entire area. The video and RFID data indicating the location and identity of each tracked animal are simultaneously sampled and stored on two computer units. (3) Video (coloured blobs) and RFID data (open circles) are then independently processed offline to extract theX–Ycoordinates of each identified mouse within the arena. The black dots represent the location of the RFID antennas. (4) The two data sets are then fused to obtain high-precision spatiotemporal tracking data. Scale bar, 10 cm. (b) A sample of 1-min trajectories of five socially interacting mice within the semi-natural arena. (c) A sample of locomotion and social behaviour classifications as extracted from 150-min trajectories of two interacting mice (as part of a group of five animals). Figure 1: Automated behavioural phenotyping system for multiple individually identifiable socially interacting animals. ( a ) Presentation of the major system components and operational stages to capture the X – Y coordinates and identification of each animal in the arena, for each processed frame. (1) Before its introduction to the enclosure, two RFID microchips (~2 mm in diameter, ~10 mm in length) are subcutaneously implanted in the ventral part of the front and hind foot of each tested animal. (2) The RFID-tagged animals are placed in a semi-natural enclosure equipped with a large central exploratory arena and eight peripheral sleeping nests. Time-synchronized video and RFID-tracking systems are used to survey the entire area. The video and RFID data indicating the location and identity of each tracked animal are simultaneously sampled and stored on two computer units. (3) Video (coloured blobs) and RFID data (open circles) are then independently processed offline to extract the X – Y coordinates of each identified mouse within the arena. The black dots represent the location of the RFID antennas. (4) The two data sets are then fused to obtain high-precision spatiotemporal tracking data. Scale bar, 10 cm. ( b ) A sample of 1-min trajectories of five socially interacting mice within the semi-natural arena. ( c ) A sample of locomotion and social behaviour classifications as extracted from 150-min trajectories of two interacting mice (as part of a group of five animals). Full size image System modules The animal-tracking apparatus consist of a custom-designed semi-natural enclosure furnished with: (1) an array of radio-frequency-identified (RFID) position-tracking system; and (2) a commercially available, standard digital video-recording unit. The tracking software was comprised two stand-alone modules: (1) an RFID-based data acquisition module and (2) a video- and RFID-tracking data fusion module (for further details see Supplementary Methods and http://www.weizmann.ac.il/neurobiology/labs/kimchi/content/downloads ). Simultaneous data collection of video and RFID data We designed a set-up for automatically tracking mouse groups within semi-natural environments for the purpose of analysing their social interactions ( Fig. 1a and Methods). The system is comprised an elaborate testing arena, of an area nearly 50-times larger than the standard laboratory mouse cage that included several shelter boxes and peripheral nest cages ( Fig. 1a , Supplementary Fig. S1 ). Such semi-natural environments have previously been demonstrated to support the monitoring of complex social interactions in mouse groups as well as improve screening quality of various behavioural alterations in mouse models [27] , [28] . The video- and RFID-tracking systems were positioned above and beneath the testing arena, respectively, to prevent any interference with the behaviour of the tested animals. The RFID-tracking device was comprised of a customized array of 39 circular antennas (~11 cm in diameter) horizontally positioned just beneath the arena floor and a standard data acquisition computer (see Methods and Supplementary Fig. S1 ). Of note, the number, size and distribution of the RFID antennas can be modified in accordance with the testing enclosure dimension (for example, for a 60 × 60 cm enclosure, only 8–10 antennas are required for tracking several mice simultaneously). The video-based tracking device was comprised of standard, commercially available, video surveillance components including a single ceiling mounted CCD video camera and digital video recording (30 fps) computer (see Methods and Supplementary Fig. S1 ). The video and RFID computers were time synchronized to allow for subsequent (off-line) tracking position data fusion ( Fig. 1a ). These fused data are then used to simultaneously and continuously track the identity and spatial position of each individual in the arena ( Fig. 1b ) as are necessary to obtain the individual and collective behavioural phenotypes ( Fig. 1c ) that are detailed below. Tracking system performance Based solely on the RFID-tracking data our system allowed the detection of the position and identity of multiple (at least ten) interacting mice with spatial resolution of about ±8–11 cm. Combining RFID- and video-tracking data significantly improved spatial accuracy to about ±0.5 cm and allowed a temporal precision of ~30 ms ( Fig. 2 and Supplementary Movie 1 ). Next we quantified the video–RFID-tracking system performance (identity and position error rate) by defining the percentage of frames in which at least two mouse identities were swapped or at least one mouse identity was not determined. We found that the system performance was 99–100% when tracking 2–3 mice simultaneously and 97–98% when tracking 4–5 mice simultaneously ( Table 1 ). When simultaneously tracking 10 mice, the percentage of identity swaps stood at ~3.5% and the overall system performance was ~94% ( Table 1 ). Notably, the identity swap rate depend only on the number of mice in the arena and number of physical interactions between pairs of mice. Conversely, it is not dependent on the experiment duration (that is, system performance is stable over time). 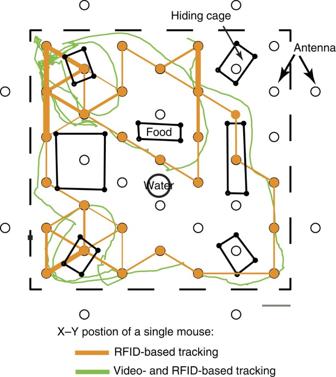Figure 2: Accuracy of spatial and identity tracking of a group of mice A representativeX–Yposition tracking of a single mouse, as extracted from the RFID-based data (orange) and from the fusion of the video- and RFID-tracking data (green). Scale bar, 10 cm. Figure 2: Accuracy of spatial and identity tracking of a group of mice A representative X – Y position tracking of a single mouse, as extracted from the RFID-based data (orange) and from the fusion of the video- and RFID-tracking data (green). Scale bar, 10 cm. Full size image Table 1 Video–RFID-tracking system performance accuracy. Full size table To further improve the accuracy of our mouse tracking analysis, we integrated our tracking software with a recently developed vision-based tracking algorithm for pairs of interacting mice (MiceProfilier [11] ). This combination further enhanced system performance by rectifying ~60% of the frames, which contained swapped identities. In a group of five mice, this is equivalent to an increase in system performance from 97.2 to 98.1%. Furthermore, integration of these two tracking systems should also yield improvements in defining the mouse-body orientation (that is, head–rear axis) which may allow characterization of more fine pairwise social behaviour phenotyping (for example, head–head investigation versus head–rear/anogenital investigation). Last, in effort to define whether the video–RFID system may be simplified, we tested what number of active RFID antennas is required to maintain high performance. We found that operating the RFID-based tracking system with 60% of the total number of RFID antennas (that is, 0.0018 antennas per cm 2 ) had only little effect on the performance. Specifically, in this case, accuracy rates were ~98% for groups of three mice (compared with >99% when all antennas are active) and ~90% for groups of six mice (compared with >95%) (for more details see Supplementary Fig. S2 ). This implies that for an arena of size 120 × 120 cm (24 times the size of conventional mouse cage)—one could use 23 antennas to get reliable tracking data. While for arena of size 60 × 60 cm only five antennas are required for reliable tracking data. System applications in phenotyping of mouse groups The integrated video–RFID system was applied to test two inbred mouse strains: C57BL/6 × 129Sv (C57 × 129) and BTBR T+ tf/J (BTBR), which were previously reported to exhibit significantly different behavioural phenotypes [29] , [30] , [31] . Three independent groups of mice were tested for each of the mouse strains (that is, a total of six experiments), using an identical standard operation protocol; the duration of each experiment was 8 days. An RFID-tagged group of five adult males, from either one of the strains, was introduced into the enclosure and the spatial position and identity of each individual were automatically identified throughout the duration of the experiment. A biologically relevant social stimulus was then presented (day 7), by introducing two alien adult female mice into the enclosure. To demonstrate the system’s behavioural phenotyping performance, three examples of data analysis are presented and discussed in details below. All analyses were performed within the same social and environmental context, but differ in that they focus on: (i) individual mouse behaviour ( Supplementary Movies 1–2 ), (ii) pair interactions ( Supplementary Movies 3–6 ), or (iii) group dynamics (social hierarchy). Individual locomotion patterns within a group To allow single-mouse behavioural analysis, we developed a set of sensitive behavioural parameters that profile an individual’s momentary locomotion patterns and its spatial position relative to key interaction–promoting objects (for example, shelter box, sleeping nest) ( Fig. 3a and Supplementary Fig. S3 and Supplementary Movie 2 ). To the best of our knowledge, this is the first report of evaluation of the locomotion/exploration behavioural phenotype of mice in the context of group social interactions and within a complex semi-natural environment. We found that, during the first 4 h of the first day ( Fig. 3b ) of the experiment, all three independently tested BTBR groups, presented a significantly lower locomotion level, that is, total distance travelled and running time percentage were lower than in the three C57 × 129 groups ( P <0.001). No significant difference was observed between the experiments within each strain. Similar findings were obtained when locomotion pattern was quantified using our RFID system alone ( Supplementary Fig. S4 ). 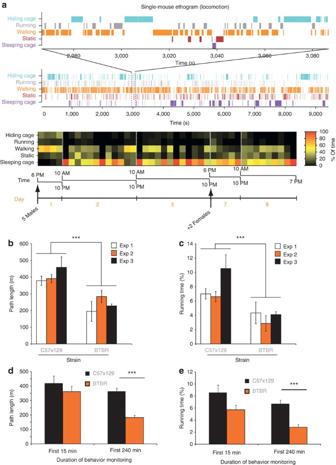Figure 3: Ethograms of five automatically detected locomotion behaviours. (a) An example of an ethogram of single-mouse locomotion features characterized by the automatically extracted trajectories and presented on three different time scales (seeSupplementary Movies 1 and 2). Upper ethogram: periods during which the mouse was engaged in each of the five examined behaviours (sleeping, hiding, static, walking and running), which are colour-coded and depicted over a period of about 2 min. The upper ethogram is a zoom-in of the middle ethogram, which represents a period of 150 min. Lower ethogram: each row corresponds to a locomotion feature, while each column represents 1 h of testing. The colour represents the percentage of time the mouse engaged in the corresponding behaviour. (b) Travelled path length and (c) percentage of running time per hour on the first day of the experiment in three independent tests (n=5 individuals for each test) in two mouse strains. (d) Travelled path length and (e) percentage of running time per hour for the first 15 min and first 240 min of testing, for two mouse strains (n=15 individuals in each strain). Data are presented as the mean±s.e.; ***P<0.001 between strains, analysis of variance (ANOVA) tests. No significant differences were detected between the experiments within each strain. Figure 3: Ethograms of five automatically detected locomotion behaviours. ( a ) An example of an ethogram of single-mouse locomotion features characterized by the automatically extracted trajectories and presented on three different time scales (see Supplementary Movies 1 and 2 ). Upper ethogram: periods during which the mouse was engaged in each of the five examined behaviours (sleeping, hiding, static, walking and running), which are colour-coded and depicted over a period of about 2 min. The upper ethogram is a zoom-in of the middle ethogram, which represents a period of 150 min. Lower ethogram: each row corresponds to a locomotion feature, while each column represents 1 h of testing. The colour represents the percentage of time the mouse engaged in the corresponding behaviour. ( b ) Travelled path length and ( c ) percentage of running time per hour on the first day of the experiment in three independent tests ( n =5 individuals for each test) in two mouse strains. ( d ) Travelled path length and ( e ) percentage of running time per hour for the first 15 min and first 240 min of testing, for two mouse strains ( n =15 individuals in each strain). Data are presented as the mean±s.e. ; *** P <0.001 between strains, analysis of variance (ANOVA) tests. No significant differences were detected between the experiments within each strain. Full size image Interestingly, evaluating the locomotion pattern during the first 15 min of the test period, a maximum testing duration of classic locomotion and anxiety-related assays (for example, open-field assay) [32] , yielded no significant behavioural difference between the strains ( Fig. 3d ). Our findings stand in line with previous studies that reported low locomotion level among BTBR mice when monitored over several hours [8] , but normal locomotion (that is, similar to other classical inbred mouse strains) when monitored over short testing duration (5–15 min) [30] , [33] . We suggest that stress-related behavioural fluctuations are reduced when testing activity patterns for extended periods of time and within semi-natural large set-ups, thereby allowing for capture of enduring behavioural phenotypes [9] , [34] , [35] . Finally, we found that five locomotion features collected by the system in a single testing day are sufficient to predict the mouse strain with an accuracy of 80–90%, the experimental stage (for example, behavioural changes upon introduction of the females) with an accuracy of ~70% and the sex with an accuracy of ~80% (see Methods and Supplementary Fig. S5 ). Social interactions between mouse pairs We developed a method for detecting and quantifying commonly observed social interactions between mouse pairs, namely, chasing/being-chased and avoidance/approach behaviours (see Methods , Fig. 4a , Supplementary Fig. S6 and Supplementary Movies 3–6 ). We found that the all-male mouse groups, from both strains, presented complex dynamic changes in pairwise social interactions over the experiment days, with the highest level of social interactions on the first day of the experiment and following the introduction of alien females to the arena (day 7) ( Fig. 4c ). Furthermore, we found that the BTBR male mice engaged in significantly fewer social interactions, when compared with the C57 × 129 male mice, throughout the experiment. This holds for analyses that address the first 15 min ( P <0.05), the first 4 h (first day) ( P <0.001, Fig. 4d ) and days 2–6 of the experiment ( P <0.001, Fig. 4e ). These findings strongly support previous studies that suggested a social behaviour deficiency in the BTBR mouse strain [29] , [31] . Moreover, we found that by using four social behaviour features collected by the system in a single testing day, we could predict the mouse strain with an accuracy of about 90–95% (see Methods and Supplementary Fig. S5 ). 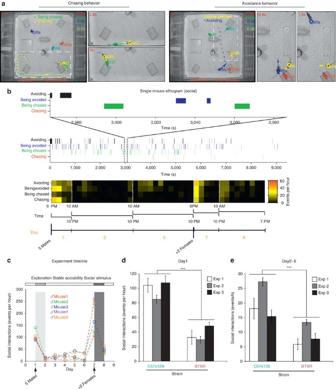Figure 4: Ethograms of four automatically detected social behaviours. (a) Sequential video frame samples of automatically detected chasing behaviour (left-hand panels) and avoidance behaviour (right-hand panels) of pairs of mice. Dashed coloured lines represent the trajectories of the socially engaged animals. Arrows represent the direction of motion for each mouse. Time codes (left upper corners) are presented relative to the first frame shown (seeSupplementary Movies 3–4). (b) Sample ethograms of four pairwise interaction features (shown for a single mouse) automatically extracted from the spatial position data and presented for three different time scales. Upper ethogram: periods during which the mouse engaged in each of the four interaction behaviours (chasing/being chased, avoiding/being avoided) are colour-coded and depicted over a period of about 2 min. The upper ethogram is a zoom-in of the middle ethogram, which represents a period of 150 min. Lower ethogram: each row corresponds to a social behaviour feature, while each column represents 1 h of testing. The colour represents the percentage of time during which the mouse was engaged in the corresponding social behaviour. (c) A representative sample of C57 × 129 mouse group social interactions over the 8 days of the experiment. On day 7 (social stimulus), two alien females were introduced into the enclosure and allowed to interact with the five resident males. (d,e) Social interaction frequency (per hour) during the first day (d) and days 2–6 (e) of the experiment. Data are presented as the mean±s.e.; ***P<0.001 between strains, analysis of variance (ANOVA) tests; no significant differences were detected between the experiments within each strain. Figure 4: Ethograms of four automatically detected social behaviours. ( a ) Sequential video frame samples of automatically detected chasing behaviour (left-hand panels) and avoidance behaviour (right-hand panels) of pairs of mice. Dashed coloured lines represent the trajectories of the socially engaged animals. Arrows represent the direction of motion for each mouse. Time codes (left upper corners) are presented relative to the first frame shown (see Supplementary Movies 3–4 ). ( b ) Sample ethograms of four pairwise interaction features (shown for a single mouse) automatically extracted from the spatial position data and presented for three different time scales. Upper ethogram: periods during which the mouse engaged in each of the four interaction behaviours (chasing/being chased, avoiding/being avoided) are colour-coded and depicted over a period of about 2 min. The upper ethogram is a zoom-in of the middle ethogram, which represents a period of 150 min. Lower ethogram: each row corresponds to a social behaviour feature, while each column represents 1 h of testing. The colour represents the percentage of time during which the mouse was engaged in the corresponding social behaviour. ( c ) A representative sample of C57 × 129 mouse group social interactions over the 8 days of the experiment. On day 7 (social stimulus), two alien females were introduced into the enclosure and allowed to interact with the five resident males. ( d , e ) Social interaction frequency (per hour) during the first day ( d ) and days 2–6 ( e ) of the experiment. Data are presented as the mean±s.e. ; *** P <0.001 between strains, analysis of variance (ANOVA) tests; no significant differences were detected between the experiments within each strain. Full size image Social hierarchy formation and stability in mouse colonies The formation of a social hierarchy is one of the most robust behavioural features presented by group-housed male mice in semi-natural conditions [36] . We developed a method to reliably define the social hierarchy rank of each individual in a group (see Methods ). Applying this analysis revealed that a clear linear-order dominance hierarchy, formed as early as the second day of the experiment and retained throughout the experiment, was evident in all C57 × 129 groups tested. Specifically, the social hierarchy of each tested C57 × 129 group consisted of a single dominant (α) and one or two sub-dominant (β) mice ( Fig. 5a and Supplementary Fig. S7 ). This stands in striking contrast to the situation in BTBR groups where almost all individuals chased each other to a similar extent and presented a weak, if any, dominant-subordinate social hierarchy pattern ( Fig. 5c and Supplementary Fig. S7 ). 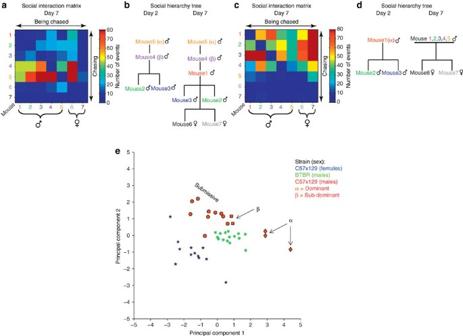Figure 5: Quantification of social dominance hierarchy of mouse groups. Social organization of a representative C57 × 129 mouse group (a,b), and BTBR mouse group (c,d). ‘Chasing’ and ‘Being-chased’ interaction matrix of a C57 × 129 (a) and BTBR group (c), on day 7 of the experiment, following a social stimulus. Colour-code at position (i,j) represents the number of events during day 7 in which mouse ‘i’ was chasing mouse ‘j’. Hierarchy trees were constructed for day 2, and day 7 of the experiment for C57 × 129 (b) and BTBR (d) groups of mice, based on the social matrices (interaction matrix not shown). Note: the social ranks of some individuals, for example, mouse 1 of the C57 × 129 group, could not be defined on day 2 due to a restricted number of social interactions; they were thus omitted from the hierarchy tree (see alsoSupplementary Fig. S7). (e) Principal component analysis was performed on all social interaction parameters gathered from day 2 until day 8 of the experiment, inclusive, in six independent experiments (red: male C57 × 129 (n=15); blue: female C57 × 129 (n=12); green: male BTBR (n=15)). Figure 5: Quantification of social dominance hierarchy of mouse groups. Social organization of a representative C57 × 129 mouse group ( a , b ), and BTBR mouse group ( c , d ). ‘Chasing’ and ‘Being-chased’ interaction matrix of a C57 × 129 ( a ) and BTBR group ( c ), on day 7 of the experiment, following a social stimulus. Colour-code at position ( i , j ) represents the number of events during day 7 in which mouse ‘ i ’ was chasing mouse ‘j’. Hierarchy trees were constructed for day 2, and day 7 of the experiment for C57 × 129 ( b ) and BTBR ( d ) groups of mice, based on the social matrices (interaction matrix not shown). Note: the social ranks of some individuals, for example, mouse 1 of the C57 × 129 group, could not be defined on day 2 due to a restricted number of social interactions; they were thus omitted from the hierarchy tree (see also Supplementary Fig. S7 ). ( e ) Principal component analysis was performed on all social interaction parameters gathered from day 2 until day 8 of the experiment, inclusive, in six independent experiments (red: male C57 × 129 ( n =15); blue: female C57 × 129 ( n =12); green: male BTBR ( n =15)). Full size image The social rank, generated by our system, of each individual within a group was validated by comparing it with the level of aggression observed in the attacks presented by tested individuals in classical resident–intruder assays [37] , [38] . The latter, manually quantified results confirmed that the dominant males identified by our automated system present the most aggressive attacks toward an alien male mouse. However, unlike our system, the classical resident–intruder assay was not spatially sensitive enough to establish the detailed social hierarchy organization within the mouse groups ( Supplementary Fig. S7 ). Furthermore, we found that integrating RFID and video data were absolutely necessary to obtain the collective behaviour phenotypes detailed below. For example, using our social interaction data in which the identities of mice are randomly swapped at some small rate leads to the complete loss of any hierarchical group structure that was present in the original data. Moreover, using our RFID system alone was insufficient for robust classification of mouse social behaviours (chasing and approaching) and group organization (see Supplementary Fig. S8 ). Finally, it should be noted that the BTBR mouse strain, unlike the C57 × 129 strain, is known to present severe socio-behavioural deficiencies and other behavioural abnormalities [30] , and is routinely used as a mouse model for studying autism [3] , [29] . This is the first time that deficiency in group social organization is reported in a mouse model for autism. This new type of social behaviour analysis may open new frontiers toward a rigorous characterization of social organizational deficiencies and an evaluation of their severity in other mouse models for autism. This report describes an animal-tracking method that enables long-term automated tracking of a large number of animals that are group-housed in elaborate semi-natural environments, while providing high temporal and spatial resolution of the identity of each individual within the group, without requiring visual tags (see Methods and Supplementary Movie 1 ). Our system is unique in that it integrates two-independent, time-synchronized position-tracking tools ( Fig. 1a ), which, when jointly applied, overcome the limitations of each single technique. For instance, a video-tracking system requires unique visual tagging (for example, painting with different colour dyes) of each animal in order to track multiple individual identities. Such visual marking is limited by the maximal number of distinguishable colour/pattern labels, has relatively high costs in terms of image analysis time and computer memory, imposes visibility constraints and may interfere with normal animal behaviour. Our use of RFID-tagging rids the system of visual markings and of limitations on the number of cohabiting animals that can be simultaneously tracked. Hence, RFID tracking provides a mean of simple, vision-independent identification of multiple individuals that may be used for classification of locomotion behavioural patterns ( Supplementary Fig. S4 ). However, the spatial accuracy of RFID tracking is substantially limited when compared with what may be achieved using video photography. Thus, using our RFID system alone was insufficient for robust classification of mouse social behaviours (chasing and approaching) and group organization ( Supplementary Fig. S8 ). Our integrated system provides a novel hybrid approach for multi-object tracking and a unique platform for both locomotion and social behaviour phenotyping of large groups of small and agile animals (for example, small rodents) ( Fig. 1 ). Moreover, as this fused tracking system is not colour-based, infra-red illumination can be used to effectively track multiple animals in the dark, which is the active period for most rodent species. As a proof of concept of the potential applications of the system towards the analysis of mouse behaviour phenotypes in complex environments and socially dynamic mouse colonies, we have developed a repertoire of user-defined analytical tools and a battery of biologically relevant parameters to characterize the locomotion and social behaviour. These enable us to robustly and consistently measure a set of behavioural traits ( Fig. 1c , Supplementary Figs S3,S4 ) that can be used to accurately classify the strain and sex of the tested animals, pairwise social interactions and social hierarchical organization ( Supplementary Fig. S5 and Fig. 5e ). Further study is required to extend our analytical toolbox to include a wider range of more subtle socio-behavioural parameters, such as sexual and aggressive behaviours, possibly by incorporating modules that allow for further analysis of our tracking data together with newly developed vision-based behavioural phenotyping programs [11] , [12] . In its current state, our system may allow rapid and systematic analysis of sets of locomotion and socio-behavioural mouse phenotypes across multiple wild-type strains and in the numerous available genetically modified models for neuropsychiatric disorders (for example, anxiety, autism and schizophrenia) [1] , [5] , [39] . Furthermore, our automated behavioural phenotyping system allows behavioural analysis over testing durations that range from several minutes (adjusted to classical testing paradigms) to a 100-fold longer (multiple hours to multiple days) within the same paradigm. Finally, as our experimental platform poses no significant size or structure constraints, it can be readily adjusted to enable a wide range of multi-purpose, stable measurements on diverse animal research models. Particularly, although not yet directly tested, our fused video- and RFID tracking technology could be applied to track the behaviour of any 2D-mobile organism (including insects, reptiles and aquatic species), so long that the animal can bear the load of an RFID tag. This may provide scientists with a means of tackling an entirely new set of questions about social behaviour across animal species and models, such as defining the mechanism underlying the formation of social hierarchy, collective group decisions and organization of large animal groups (for example, insect colonies, fish schools) [40] . Animals Adult male and female mice from the C57BL/6Jx129sv and BTBR T<+> tf/J strains (both from Jackson Laboratories, ME) were used in the experiments. Mice were housed and bred in a pathogen-free animal facility on a 12/12 h light/dark cycle, with food and water ad libitum . All experimental procedures were approved by the IACUC of the Weizmann Institute of Science. RFID-based mouse tagging Two RFID microchips (ID-100, operating frequency 125–135 kHz; Trovan Ltd) were subcutaneously implanted into anaesthetized mice, 2 weeks before the initiation of the experiment. We found that for best detection of RFID signals, the microchip should be positioned perpendicular to the RFID antennas, which lay horizontally beneath the enclosure floor. Hence, to achieve best signal intensity by the RFID antennas, the microchips were implanted lengthwise beneath the skin, parallel to the lower hind/front limb of the mouse. We confirmed that the implanted microchips did not interfere with the health or typical behaviour of the mice for at least 6 months following implantation. Testing procedure Each experiment tested seven adult mice of the same age and strain. On day 1 of the experiment, five non-littermate males were introduced in random order into the enclosure. On day 7, two alien adult females were introduced into the enclosure and allowed to socially interact with the five males. On day 8, the experiment was terminated. On day 8, all mice were removed from the enclosure. The males were housed individually in a cage for 1 week and then tested in a classical resident–intruder assay, by exposing each individual to an alien male mouse and manually evaluating the resident mouse’s social behaviour (for example, aggression) toward the alien mouse, as previously described [38] . The manually recorded aggressive behaviour of the resident males toward the alien mouse was compared with the automatically quantified behaviour ( Supplementary Fig. S7 ). Experimental set-up Enclosure : The testing enclosure included a large central square exploratory arena (L × W × H, 119.2 × 119.2 × 80 cm) constructed of transparent polycarbonate boards. In addition, two standard mouse cages were fitted to each of the four arena walls by short Perspex tubes, and served as sleeping nests. Mice were allowed to freely move between the exploratory region and the sleeping nests. The arena floor was covered evenly with sawdust bedding. It was also equipped with custom-made transparent shelter boxes and bridges, as well as with a custom-made, free-access feeder (rodent pellets) and water container ( Supplementary Methods and Supplementary Fig. S1 ). RFID position-tracking system : The tracking system was comprised the following parts: (1) an array of antennas; (2) RFID decoder cards (LID650; Trovan Ltd); and (3) a PC equipped with an RS485 data acquisition card PCIe-8431/8 (National Instruments). The 39-antenna array was positioned beneath the floor of the exploratory arena (4–5 cm beneath the bedding surface) and one antenna was positioned beneath each of the eight tubes connecting the peripheral cages with the exploratory arena ( Supplementary Fig. S1 ). Uniquely identifiable RFID decoder cards, with a reading rate of 24 ms, were connected to each antenna in the array and transmitted their data to the PC. Video position-tracking system : A low-light sensitivity, black and white CCD camera (MTV-13V5HC Mintron; 795 × 596 pixels) and infra-red LED illuminators were mounted above the arena to allow video recording of mice behaviour in the arena throughout both day and night. Video data were recorded on a commercial multi-channel digital video recording computer (DVR; CTTI Ltd) that allows video-recording from multiple cameras, at 30 frames per second. Time-synchronization of RFID and video recording computers : High-accuracy time synchronization is essential for system operation, and was achieved using Absolute Time Server software (FlexibleSoft) installed on both the video- and RFID-recording computers. The DVR computer was set to serve as the ‘time server’ (the time setter of the experiment) and the RFID-recording computer was configured to serve as the ‘time client’ computer. Video and RFID-based trajectory extraction Our software is comprised several stand-alone software modules ( Supplementary Methods ), as listed below. RFID-based data acquisition software : The RFID-acquired spatial position data of each mouse were recorded using a software module we wrote in Lab Windows/CVI (see Supplementary Methods ). The software was designed to instantly extract the information transferred to the RFID decoders each time a mouse crossed/stood above one of the RFID antennas. Our software recorded the following parameters: the 10-digit number of the detected RFID microchip, the antenna/decoder number by which it was detected, and the date and time (with a resolution of 1 μs). The data were stored locally on the RFID-recording computer (see Supplementary Movie 7 ). Video-based mouse location extraction : We used OpenCV C++ to write software to determine (off-line) the spatial position of each mouse in each recorded video image frame. The software extracted the location of each mouse in a four-step process ( Fig. 1 ). (1) The background was subtracted from each video frame. (2) The pixels belonging to each mouse in the arena were determined. (3) The video pixels for each mouse detected in the exploratory arena were clustered using k-means clustering. (4) The X – Y position of each mouse was extracted by computing the center of mass of each of the clustered pixels (see Supplementary Methods ). System performance and error rate analysis : Tracking system performance was automatically analysed using a Matlab application designed for this purpose and was validated by two well-trained human observers. We analysed tracking accuracy over several hours of recordings, from three independent experiments, as a function of the number of mice detected in arena during the testing duration ( Table 1 ). The system performance index was defined as the percentage of the recorded video frames in which the tracked mice were successfully identified and localized. This was defined as: 100−(swap identities+unknowns) (%). Swap identity was defined as identity of swapping/jumping to a wrong location limited by ~4 cm offset. Unknown was defined as mouse identity and localization that could not be identified. Quantification of behavioural parameters Locomotion behavioural parameters : Locomotion and social interaction behaviours were extracted for each mouse from the trajectory data. The locomotive behavioural pattern assessed the following five parameters ( Fig. 3 and Supplementary Movie 2 ): ‘Sleeping (nest) cage’—the spatial position of the mouse was within one of the peripheral sleeping cages. ‘Hiding cage’—mouse spatial position was within one of the arena’s shelter cages. ‘Static’—the mouse was stationary (speed: <1 cm s −1 ) in the exploratory arena. ‘Walking’—the mouse was moving in the arena with a mean speed within given ranges. ‘Running’—the mouse was moving in the arena at a mean speed, which exceeded the maximum speed of walking (see Supplementary Methods ). The speed ranges were set based on examples of previously reported physical measurements of laboratory mice [41] , [42] . Social behavioural parameters : Socio-behavioural patterns between a pair of mice (Mouse A and Mouse B) measured the following parameters: chasing/being chased and avoiding/being avoided ( Fig. 4 , Supplementary Movies 3–6 and Supplementary Methods ). In brief, chasing behaviour was defined as follows: Mouse A running after Mouse B was defined as the ‘chasing’ mouse, while mouse B was defined as the ‘being chased’ mouse. Behaviour was classified as chasing when two mice were moving forward in the same direction and time, the two interacting mice travelled at least 60 cm, the distance between the two mice was below 40 cm, and the trajectory correlation between the interacting mice was >0.7. Avoidance behaviour was defined as follows: Mouse A advanced toward Mouse B (which was walking or static), which led Mouse B (the ‘avoiding mouse’ to rapidly change direction and flee from Mouse A (the ‘being avoided’ or ‘approaching’ mouse (see Supplementary Methods ). Validation of social behaviour parameter classifiers : The data analysis software for classification of social behaviour patterns was evaluated by comparing the machine quantification results with those derived from manual quantification by two trained human observers. We found that for classifying of ‘no social interaction’, the evaluation provided by our automated classifier was in full agreement with the quantification of both human observers. Surprisingly, we revealed that developing classifiers to distinguish between types of social interactions (in particularly of avoidance behaviour) is an extremely challenging task as even well-trained human observers will often disagree with regard to correct classification of behaviour (that is, the ground truth). Our automatic classifier was at least as good as either one of the well-trained human observers for classification of chasing and avoidance behaviour ( Supplementary Fig. S9 ). Social hierarchy status : A social hierarchy tree for each mouse group (five males and two females) was constructed based on the chasing/being-chased pairwise interaction data for each day of the experiment ( Fig. 5 ). First, the pairwise relationships between the mice (dominant-subordinate, equality or undetermined) were classified [43] . The classification was based on comparing the number of wins (in chasing events) with the total number of chasing/being chased interactions. In the case of a conflict in determining the social ranks (that is, A>B, B>C, C>A), the animal hierarchy was defined as undetermined. How to cite this article: Weissbrod, A. et al . Automated long-term tracking and social behavioural phenotyping of animal colonies within a semi-natural environment. Nat. Commun. 4:2018 doi: 10.1038/ncomms3018 (2013).